An exact arithmetic toolbox for a consistent and reproducible structural analysis of metabolic network models Constraint-based models are currently the only methodology that allows the study of metabolism at the whole-genome scale. Flux balance analysis is commonly used to analyse constraint-based models. Curiously, the results of this analysis vary with the software being run, a situation that we show can be remedied by using exact rather than floating-point arithmetic. Here we introduce MONGOOSE, a toolbox for analysing the structure of constraint-based metabolic models in exact arithmetic. We apply MONGOOSE to the analysis of 98 existing metabolic network models and find that the biomass reaction is surprisingly blocked (unable to sustain non-zero flux) in nearly half of them. We propose a principled approach for unblocking these reactions and extend it to the problems of identifying essential and synthetic lethal reactions and minimal media. Our structural insights enable a systematic study of constraint-based metabolic models, yielding a deeper understanding of their possibilities and limitations. Flux balance analysis (FBA) [1] , [2] , [3] , [4] , [5] , [6] has been the dominant approach to analysing constraint-based metabolic network models, as an alternative to mass-action kinetic models [7] and biochemical systems analysis [8] that cannot currently be performed on a whole-genome scale. This analysis of metabolic network models typically reveals a number of key structural elements. It allows the identification of blocked reactions, which are reactions that cannot have a non-zero flux due to the constraints of the model [9] , as well as enzyme subsets, which are groups of reactions constrained to have proportional fluxes to one another [10] . FBA leads to predictions about the growth rate of a cell under various conditions defined by the availability of specific nutrients [5] , the minimal media, smallest sets of nutrients allowing growth [11] , essential genes [12] and synthetic lethal reactions [13] , groups of one or two reactions whose deletion is predicted to disable growth altogether. Most previously published tools for FBA use floating-point arithmetic [14] . Here, we argue that performing FBA in floating-point arithmetic may lead to inconsistent and occasionally irreproducible analysis results. These arise because floating-point arithmetic is designed to provide a correct answer to a question about a slightly perturbed version of the input, which makes sense in most applications, but not metabolic network analysis. Indeed, since the stoichiometric coefficients are small integers or ratios of such integers, the perturbed version of the input does not correspond to a valid model. In other words, floating-point arithmetic does not provide a mechanism for ensuring that the constraints of the model are satisfied exactly, rather than within a small tolerance. Moreover, while previously published tools perform some structural analysis of the input model, there are several features that these analyses tend to lack. First, the blockage of a reaction in the model is usually remedied by the addition of one or more reactions from a database of biochemical reactions [15] , even though the blockage may also be due to incorrect irreversibility constraints on the reactions in the model, an idea that has only been explored sporadically [16] . Second, the fact that some reversible reactions are able to proceed in only one of the two possible directions due to model constraints, suggesting a discrepancy between model functionality and biological assumptions, has not been recognized in previous analyses. Last, the structural analysis was not guaranteed to stop after a single cycle, proceeding instead over multiple iterations [10] . We address these limitations by introducing the MONGOOSE (MetabOlic Network GrOwth Optimization Solved Exactly) toolbox. Its core is an exact arithmetic-based algorithmic pipeline ( Fig. 1 ) which incorporates a structural analysis supported by new theoretical results. In particular, MONGOOSE classifies each blocked reaction into one of three categories based on the cause of blockage, and proposes small sets of constraints that can be relaxed to remove the blockage. The toolbox also identifies semiblocked reactions, those reversible reactions in which one of the two possible directions is blocked and similarly proposes ways of unblocking them. In addition, the structural analysis performed by MONGOOSE is proven to converge after a single cycle and allows the user to perform further analyses like the identification of minimal media, essential genes or synthetic lethal reactions on a significantly smaller model. 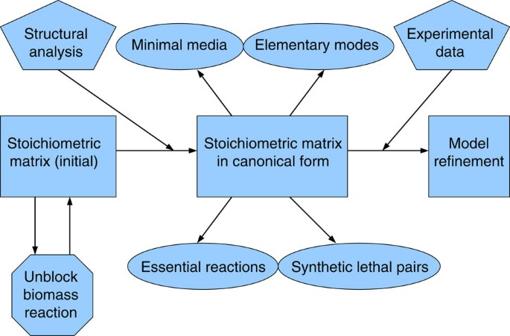Figure 1: Flowchart of the MONGOOSE pipeline. A schematic representation of the interaction between different parts of the MONGOOSE pipeline. Figure 1: Flowchart of the MONGOOSE pipeline. A schematic representation of the interaction between different parts of the MONGOOSE pipeline. Full size image We apply MONGOOSE to the 98 genome-scale metabolic network reconstructions collected in the UCSD Systems Biology repository [17] . We show significant differences between the results of MONGOOSE and COBRA [14] , a widely used toolkit for metabolic network analysis, and produce independently verifiable correctness certificates for those of MONGOOSE. Furthermore, we surprisingly find that of the 89 networks with a well-defined biomass reaction, 44 cannot exhibit in silico growth under any condition (are blocked). MONGOOSE provides a detailed diagnosis of the reason for this situation by identifying a small set of constraints whose relaxation resolves the blockage. Our toolbox also identifies all essential and synthetic lethal reactions and defines minimal media [11] , problems for which MONGOOSE provides the additional benefit of a dramatic lossless compression of the metabolic network, similar in spirit to the use of compressive methods in genomics [18] . This compression allows the complete analysis of all 98 models to finish in less than one day. MONGOOSE thus produces certifiably consistent and reproducible results, while leveraging its structural insights to convert many previously intractable problems in metabolic network analysis, including those involving energy balance analysis, to more tractable ones. Finally, MONGOOSE provides a module for checking the correctness of any flux mode or cutset (set of reactions whose deletion disables growth) in exact arithmetic. The software implementing MONGOOSE is freely available at http://mongoose.csail.mit.edu/ , and also as Supplementary Software. Overview of the MONGOOSE pipeline The MONGOOSE pipeline is designed to perform a complete structural analysis and reduction of a metabolic network. Previous methods, such as the approach introduced by Gagneur and Klamt [10] , were able to perform such analysis as well, but this analysis was substantially less complete than the one we present here. In particular, MONGOOSE provides a more detailed classification of blocked reactions, identifies semiblocked reactions, groups together all the enzyme subsets, and converges in a single iteration instead of multiple ones. If the biomass reaction is blocked, MONGOOSE can unblock it by relaxing a small number of constraints. Importantly, the structural analysis results in the reduction of the metabolic network model to a smaller model which preserves all the information contained in it. The reduced metabolic network can then be used to efficiently identify essential and synthetic lethal reactions and minimal growth media. The complete pipeline is illustrated in Fig. 1 and described in more detail in the Methods, where the structural features identified by MONGOOSE are demonstrated on a small example from the MetaTool website [19] , augmented with an additional seven metabolites and 10 reactions for illustration purposes. An additional illustration of structural features identified by MONGOOSE is provided in Supplementary Figure 1 . In addition to the more extensive structural analysis, a key distinguishing feature of MONGOOSE is its use of exact arithmetic. This ensures that a certificate is produced for each feature which can be verified independently of the analysis. Such a certificate may consist, for instance, of the coefficients of a linear combination of the model constraints that imply that a particular reaction is blocked (cannot have a non-zero flux), or that two reactions in an enzyme subset always have fluxes that are proportional to one another. Existence of these certificates and an effective way of producing them are guaranteed by the theoretical results in Supplementary Notes 1–8 . MONGOOSE identifies novel structural features Unlike previous work [14] , [20] , where blocked reactions are identified regardless of the cause of blockage (with the possible exception of dead ends, reactions which contain a unique internal metabolite [14] ), MONGOOSE distinguishes between three kinds of blocked reactions. We further introduce two kinds of semiblocked reactions, that is, reversible reactions which only admit flux in one of the directions, a feature that, to the best of our knowledge, has not been identified in earlier work. For each topology-blocked reaction (one whose blockage follows from the topology of the metabolic network), MONGOOSE returns an informative causal chain leading to the identification of the blockage, which helps remove the blockage in many cases. For each stoichiometry-blocked reaction i , MONGOOSE can identify a linear combination of the metabolites that contains a 1 in position i and a 0 everywhere else; the structural result we prove in Supplementary Note 2 shows that there is always such a linear combination. For each irreversibility-blocked reaction i , MONGOOSE can identify a subset of irreversible reactions that is responsible for the blockage. For each semiblocked reaction i , MONGOOSE can identify a subset of the constraints that is responsible for the semiblockage. It also labels semiblocked reactions as irreversible and reverses the direction of the effectively reverse ones by multiplying their stoichiometric coefficients by –1. In addition to deleting all blocked reactions and adjusting semiblocked reactions to be irreversible, MONGOOSE groups reactions that always have proportional fluxes into enzyme subsets, using a previously described method [10] , which we show in Supplementary Note 5 to be sufficient to identify all such subsets. This process reduces the size of the model without losing any information. As a final step, MONGOOSE identifies and removes a maximal set of redundant flux balance constraints, those that can be created from the remaining ones by taking linear combinations. This reduction sets the stage for further analyses, such as the identification of essential and synthetic lethal reactions and of minimal media. Consistency and reproducibility require exact arithmetic A fundamental question in constraint-based metabolic network models is whether a particular reaction can be active under given environmental conditions (growth media). Biochemical reactions, and therefore stoichiometric matrices, have rational coefficients. In fact, except for a small number of reactions involving cofactors, most of these coefficients tend to be small integers. Since the constraints on a metabolic network are represented through its stoichiometric matrix, it is critical that this representation be accurate. However, the linear programming solvers typically used in metabolic network analysis represent the entries of stoichiometric matrices as floating-point numbers, leading to a marginal loss of accuracy. While such loss of accuracy is acceptable in many applications, issues resulting from it have been attested to in the context of integer programs, which use the results of linear programs to make branching decisions in a branch-and-bound approach [21] . Our experience also shows this accuracy loss to be a problem for metabolic network analysis. Indeed, it is not sufficient to know whether a slightly perturbed version of a metabolic network can have a non-zero flux through a given reaction because this knowledge gives no information about whether this condition is true for the actual network. This argument implies that backward stability, the usual requirement for numerical linear algebra algorithms [22] , is not sufficient for metabolic network analysis, and forward stability (the right answer for the actual network) is needed. In addition, our theoretical results, proven in Supplementary Notes 1–8 , break down in floating-point arithmetic and only hold in exact arithmetic. For this reason we implement all our algorithms in exact arithmetic and perform all our linear optimizations using the QSopt_ex solver [23] . One major advantage of using this solver is that it provides a certificate for the correctness of the solution to a linear optimization problem, meaning that its results can be verified independently of the solver. This ability is to be contrasted with an almost exclusive use of floating-point-based linear program solvers in the field of metabolic network analysis today, which only provide approximate certificates and whose solutions are only approximately correct. While some existing approaches, such as the MetaTool toolbox [19] , do use exact arithmetic, their application to the analysis of genome-scale metabolic networks is mostly restricted to elementary mode enumeration. Instead of using exact arithmetic, one could attempt to compute the tolerance required to guarantee an exact solution based on the input stoichiometric matrix. Unfortunately, as we discuss in the Methods, this computation turns out to be difficult in its own right, while approximating the tolerance from below gives extremely small values that would make the calculation of a solution prohibitive. The results of MONGOOSE reveal inconsistencies in COBRA To certify that exact arithmetic gives different results from floating-point arithmetic in practice, we compared our results with those produced by the popular COBRA toolbox [14] . Under default settings, COBRA successfully parsed 30 models out of the 98 models we investigated. Both COBRA and MONGOOSE detected a well-defined biomass reaction in 17 of these 30 network models. In terms of deciding whether the biomass reaction is blocked, there were multiple discrepancies between COBRA and MONGOOSE. Specifically, three of the models—the Escherichia coli iAF1260, Helicobacter pylori iIT341 and Mycobacterium tuberculosis iNJ661—were predicted to be able to grow by COBRA, but not by MONGOOSE. This difference is due to COBRA not enforcing the flux balance constraints on internal metabolites exactly—even if the deviations from exact flux balance are small, they can make the difference between a feasible and an infeasible problem. Similarly, significant differences were identified between the total numbers of blocked reactions predicted by COBRA and by MONGOOSE. The differences did not all go in the same direction. For instance, in the Escherichia coli iJO1366 model, COBRA and MONGOOSE respectively found 878 and 639 blocked reactions out of a total 2,583, while in the Saccharomyces cerevisiae iND750 model, they respectively found 635 and 796 blocked reactions out of a total 1,266. These discrepancies clearly show that the floating-point approach differs from the exact arithmetic approach not only in theory, but also in important practical cases. To further investigate the discrepancy between the floating-point and the exact arithmetic analyses, we extracted the smallest of the models, the Helicobacter pylori iIT341, predicted not to be able to grow by MONGOOSE, into a 363 × 461 stoichiometric matrix which we then submitted to the various solvers available at NEOS [24] to optimize its growth rate in rich media. Out of six linear programming solvers on NEOS, five predicted a non-zero growth rate, and only CPLEX [25] predicted a zero growth rate, in agreement with QSopt_ex used by MONGOOSE. This result suggests that a toolbox like COBRA is highly sensitive to the particular floating-point solver it uses and will be unlikely to predict the status of the biomass reaction correctly in a large genome-scale metabolic network unless it uses a solver such as CPLEX [25] , which has the stringent feasibility tolerance (maximum allowed violation of a constraint in a linear program) of 10 −6 as its default value. However, even in case the feasibility tolerance is set to the smallest allowed value of 10 −9 , rounding errors lead to the failure of identifying many pairs of reactions as belonging to the same enzyme subset, as we show in Fig. 2 and describe in detail in the Methods; thus the use of an exact arithmetic solver, like QSOpt_ex used in MONGOOSE, is justified. 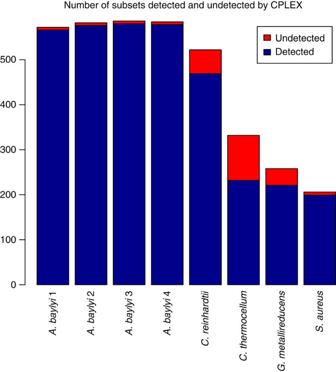Figure 2: Comparison of CPLEX and MONGOOSE. MONGOOSE identifies all reaction pairs that are in an enzyme subset for these eight metabolic networks. The reaction pairs detected as being in an enzyme subset by CPLEX are shown in blue, while those not detected as such are shown in red. Figure 2: Comparison of CPLEX and MONGOOSE. MONGOOSE identifies all reaction pairs that are in an enzyme subset for these eight metabolic networks. The reaction pairs detected as being in an enzyme subset by CPLEX are shown in blue, while those not detected as such are shown in red. Full size image To make it easier for users of other toolboxes, such as COBRA [14] or CellNetAnalyzer [20] , to verify the correctness of the results they obtain, we also provide a module in MONGOOSE which can either validate or correct these external computation results by using exact arithmetic. To do so, it suffices to provide MONGOOSE with a description of the metabolic network and a description of the flux vector or cutset produced by the external software. For flux modes, MONGOOSE computes the distance from the given vector to the flux cone determined by the model, and either validates the result if this distance is 0, or produces the flux mode closest to the given one if it is not. For cutsets, MONGOOSE checks whether the set of reactions indeed forms a cutset for the reaction of interest, and if it does not, finds a small additional set of reactions that can be added to it to form a cutset. The biomass reaction is blocked in 44 out of 89 models When MONGOOSE is run on previously published models ( Supplementary Table 1 ), the most striking feature is the fact that 44 out of the 89 models containing a well-defined biomass reaction cannot exhibit growth without the additional modifications discussed below. The fact that this result had not been discovered before is due to our novel use of exact arithmetic for the genome-scale analysis. This finding likely indicates that the current state of our knowledge of metabolism may be less complete than thought, and illustrates the sensitivity of constraint-based models to the particular coefficients used to reflect the biomass composition. Overall, very small perturbations to the coefficients of a biomass reaction are typically insufficient to enable growth ( Supplementary Note 8 ). However, the smallest perturbation required to be made to the coefficients of the biomass reaction, defined as the smallest δ such that changing all biomass coefficients by values at most δ enables growth, varies substantially across the blocked models we investigated, from one as small as 3 × 10 −8 for the iIN800 model of Saccharomyces cerevisiae to 5.3 for a model of Staphylococcus aureus . These values are shown in the last column of Supplementary Table 1 . This finding suggests that in a few models, making small changes to the biomass coefficients is indeed sufficient to remove the blockages, while in the majority of models, further modifications may be required. MONGOOSE diagnoses blockages and proposes ways to remedy them MONGOOSE also diagnoses the underlying cause of blockage and proposes possible solutions. MONGOOSE distinguishes between three types of blocked reactions (further discussed in the Methods). Often, a topology-blocked biomass reaction can be resolved immediately by either adding a biomass export reaction or treating the biomass metabolite as external, or correcting obvious typographical errors in the model. These approaches resolve the problem for 23 out of the 33 topology-blocked models (highlighted in yellow in Supplementary Table 1 ), with 11 actually being able to produce biomass after the correction and the rest being blocked for the more complicated reasons described below. Furthermore, many models do not contain a proper specification of external metabolites, or have incorrectly compartmentalized transport reactions. We correct all of these models and unblock three out of the five that were previously blocked. All these models are highlighted in blue in Supplementary Table 1 . In addition to being topology–blocked, the biomass reaction can be stoichiometry or irreversibility–blocked. For the first type of blockage, our approach relaxes some balance constraints on internal metabolites, allowing them not to be perfectly balanced; for the second type of blockage, it relaxes some directionality constraints on irreversible reactions, allowing them to proceed in the reverse direction. We find that all the 44 models which cannot exhibit growth can be unblocked by relaxing an average of five constraints ( Supplementary Table 1 ). MONGOOSE finds other blocked reactions and enzyme subsets In addition to the biomass reaction being blocked in many of the models we investigated, most of them have a large fraction of other blocked reactions. This fraction varies from 3.8% for Buchnera aphidicola to 95.1% for Pichia pastoris PpaMBEL1254, with an average of 36.3%. As with blocked biomass reactions, this situation suggests gaps in the current state of our knowledge of metabolism. All semiblocked reactions (ones for which only one direction is effectively possible) are converted to be irreversible, and effectively reverse ones are flipped (multiplied by –1). We find that up to 30% of all unblocked reactions are effectively forward, and up to 20% of all unblocked reactions are effectively reverse, with the maximal values reached by Rhodobacter sphaeroides and Pichia pastoris PpaMBEL1254, respectively. The average fractions of effectively forward and effectively reverse reactions are 12.0% and 5.5%, respectively. We find that a significant fraction of the unblocked reactions in each network is part of an enzyme subset (reactions whose fluxes are constrained to be proportional to one another). This fraction varies from 16.0% for Aspergillus nidulans to 91.8% for Pichia pastoris PpaMBEL1254, with an average of 53.2%. The biomass reaction is in an enzyme subset when it is not blocked in all but five of the models, possibly because of the large number of metabolites (and hence constraints) it typically involves. MONGOOSE identifies small reaction cutsets and minimal media A reaction cutset is a set of reactions whose deletion disables growth by forcing the flux through the growth reaction to be 0. A cutset containing only one reaction is called an essential reaction. An essential reaction is thus one which is indispensable for biomass production in silico (since we do not constrain the fluxes through exchange reactions, this corresponds to essentiality for growth in a rich medium). This definition of essentiality is identical to the one used in early work on constraint-based models [26] as well as more recently in ref. 27 , but differs from non-standard topological approaches [6] and the flux surplus rather than flux balance model [28] . In addition to those reactions which are in an enzyme subset with the biomass reaction, there may be other reactions that are essential. We find that up to 77.2% (for Buchnera aphidicola ) of all unblocked reactions not in an enzyme subset with the biomass reaction are essential, with an average of 9.7%. A cutset containing two reactions neither of which is essential is called a synthetic lethal pair. We find that up to 9.7% (for Buchnera aphidicola ) of all unblocked nonessential reaction pairs are synthetic lethal, with an average of 0.31%. A minimal medium is a smallest set of exchange reactions that is sufficient for the organism to produce biomass [11] . While the MONGOOSE pipeline cannot find the smallest set of such reactions (this is a computationally intractable problem in general [12] ), it is able to find small minimal media for all the organisms with an unblocked biomass reaction. The size of the smallest minimal medium ranges between 1 and 43 exchange reactions, with an average of 10. MONGOOSE significantly reduces the size of the networks A remarkable result of applying the MONGOOSE pipeline is that the resulting stoichiometric matrix is significantly smaller than the original stoichiometric matrix, providing an average 4.2-fold reduction in the number of reactions. This reduction in size varies from a factor of 1.35 for the metabolic network of Saccharomyces cerevisiae iLL672 to a factor of 139 for Pichia pastoris PpaMBEL1254. We reduce a stoichiometric matrix by observing that blocked reactions do not contribute to the metabolic capabilities of the model; enzyme subsets can be combined into single reactions without loss of information; and redundant constraints do not change a model’s behaviour. We say that a stoichiometric matrix is in canonical form if it contains no blocked reactions, enzyme subsets or redundant constraints, and show ( Supplementary Note 6 ) that the proposed reduction process finishes after a single iteration because the reduced network is guaranteed to not contain any of these structural elements. MONGOOSE applies energy balance analysis to reduced networks Energy balance analysis [29] , [30] , [31] provides an additional set of constraints on possible flux vectors to ensure that they are consistent with the laws of thermodynamics. These constraints require, for each admissible flux vector v , an energy vector w in the row space of the part of the stoichiometric matrix S containing internal reactions whose entries have signs opposite to the corresponding entries of v . We consider weakly feasible flux vectors (called T-feasible vectors in ref. 30 ) by allowing w to have non-zeros where v has zeros, but not vice versa (equation (2)). We can apply the same theoretical results that we used to structurally analyse and reduce the stoichiometric matrix S to energy balance analysis, which allows us to identify several structural features. Enzyme subsets that contain only internal reactions and add up to a reaction with all coefficients equal to 0 are blocked, because any energy vector would have to have a 0 in the position corresponding to such a reaction, therefore constraining its flux to 0 as well. Such reactions, which we call zero loops, are a special case of type III loops [31] . The fraction of enzyme subsets that are zero loops reached 55.0% for Pichia pastoris PpaMBEL1254, with an average of 1.7%. In addition to zero loops, energy-blocked reactions can be identified from the irreversibility constraints, when the requirement that implies that w i =0 and hence v i =0. The fraction of energy-blocked reactions after the deletion of zero loops reached 88.3% for the Buchnera aphidicola model, with an average of 6.4%. Energy balance analysis also allows us to identify unidirectional reactions (analogous to the semiblocked reactions), reversible reactions which only have one possible direction due to the energy balance constraints. The fraction of unblocked reactions that were effectively reverse due to energy balance constraints reached a maximum of 11.3% for Chromohalobacter salexigens , with an average of 1.1%. Surprisingly, there were no effectively forward reactions due to energy balance constraints in any of the models. Additionally, any isozymes (reactions that are multiples of one another) can be grouped into a single isozyme subset for the purpose of energy balance analysis, as their energy vectors are constrained to have proportional values; they are analogous to the enzyme subsets deduced from the flux balance constraints. The fraction of unblocked internal reactions in an isozyme subset reached 85.1% for Methanosarcina acetivorans iMB745, with an average of 16.8%. All the model-specific results are displayed in Supplementary Table 1 . Because the constraints imposed by energy balance are nonlinear, the reductions obtained by using them lead to further reductions due to the flux balance constraints. For this reason, MONGOOSE alternates between the reductions due to energy balance and flux balance until no further changes can be made due to either one. This requires an average of six iterations. After this process terminates, the growth reaction ends up being blocked due to the combined effect of flux balance and energy balance constraints in 30 out of 59 models where it is not blocked due to flux balance constraints alone (we indicate this as ‘EnergyBlocked’ in the GrowStatus column in Supplementary Table 1 ). In additon, the final network is significantly smaller than the initial reduced network. The reduction in size varies from a factor of 1.01 for Shewanella oneidensis to 68 for Buchnera aphidicola , with an average reduction factor of 2.33. MONGOOSE exhibits a reasonable running time While the exact arithmetic approach used by MONGOOSE necessarily slows down the computations, in our experience, the slowdown never exceeds an order of magnitude. Thus, the complete structural analysis of all 98 metabolic network models required a total of only 10 h of processing on a single processor. This corresponds to an average of 6 min per metabolic network model. In comparison, the COBRA toolbox [14] required, on average, just under a minute to find the blocked reactions based on flux variability analysis in a metabolic network, with the average computed over the networks it was able to parse directly. COBRA does not appear to identify enzyme subsets directly, only to find correlated sets of fluxes based on a sample of flux vectors from the model, which appears sufficiently different from our task to justify excluding it from the comparison. This small decrease in speed is, however, more than compensated for by the reproducibility and robustness of the results, as well as the significant reduction of the size of the metabolic network that speeds up all subsequent analyses. In particular, the complete identification of all essential reactions and synthetic lethal pairs in the 56 models with a well-defined biomass reaction that was not blocked required a total of 5 h of additional processing time, or less than 6 min per metabolic model, using the search algorithm described in Methods. The iterative application of energy and flux balance to the reduced networks required an additional 12.5 h. We asserted that while constraint-based metabolic network models are a valuable tool for gaining insight into metabolism, their analysis needs to be done in exact arithmetic to ensure that their results are consistent and reproducible. The fact that MONGOOSE revealed that 44 out of 89 previously published networks containing biomass reactions cannot exhibit in silico growth may point to the need for more complete network reconstructions or, more likely, to the need for a more accurate measurement of biomass coefficients. Our work provides several important contributions to the field of metabolic network analysis. On the theoretical front, MONGOOSE is grounded in a solid theoretical basis consisting of novel results about the structure of constraint-based genome-scale metabolic network models. Furthermore, to the best of our knowledge, the need for using exact arithmetic in metabolic network analysis has never been explicitly demonstrated on a large collection of existing genome-scale metabolic network models, as we have done using MONGOOSE. On the practical front, MONGOOSE makes three key contributions. First, it is able to perform a complete structural analysis of the network as a preprocessing step, providing useful insights into possible sources of incompleteness and identifying and troubleshooting any issues leading to the blockage of the growth (biomass) reaction. Second, MONGOOSE substantially compresses the metabolic network, making it more feasible to perform further analyses (gene essentiality, synthetic lethality, minimal media and some energy balance analysis) without losing any information. Third, MONGOOSE provides an automated interface that parses the network, translates the problem into a format suitable for any linear programming solver and parses the solution returned by the solver into a format suitable for further processing, as well as a module for checking the validity of flux vectors and cutsets obtained by any other solver in exact arithmetic. All these features can be readily integrated with existing pipelines for metabolic network analysis. An approach based on our theoretical results could also be used to identify some or all elementary flux modes [12] and minimal cutsets [13] in a metabolic network, as discovered independently by another research group [32] . Future work could also include more fully incorporating energy balance constraints into the analysis, as well as making use of additional information, such as the Gibbs’ free energy of reactions, to further constrain the problem, along the lines of refs 16 , 33 , 34 . Additional refinements could include restricting the proposed changes to metabolic networks with blocked growth based on biological knowledge, such as not allowing certain reactions to proceed in the reverse direction when unblocking irreversibility blockages. Our primary focus has been on identifying potential model inaccuracies as opposed to prediction, because we believe that a faithful representation of the philosophy of constraint-based modelling coupled with reliability and reproducibility of results has a higher priority than predictive power. If any existing models are designed in such a way that the inaccuracies in them cancel out the errors introduced by floating-point arithmetic to produce good agreement with experimental results, reversing the effect of floating-point errors may temporarily result in a decrease of predictive power, but only until model inaccuracies are corrected in turn. In the future, we plan to combine our analysis efforts with comparing predictions to experimental data. The joint efforts of model developers and analysis tool developers will ultimately result in models with high predictive power under a robust analysis method. We believe that the exact arithmetic approach to the analysis of constraint-based metabolic networks opens a number of new possibilities in metabolic network analysis. First, the genome-scale metabolic network reconstructions with blocked biomass reactions can be completed or their coefficients measured more accurately. Second, the MONGOOSE methodology may be used to reconcile the predictions of metabolic network models with experimental data, leading to further refinement. Finally, MONGOOSE can be used to support genome-scale network reconstruction by helping the modeller identify incompletely reconstructed pathways or unexpected features that can be resolved experimentally. We are currently engaged in a project of this type focusing on the reconstruction of a metabolic network model for Bordetella pertussis . It is our hope that the community will adopt the MONGOOSE software as the basis for further development of metabolic network analysis methods. This section is organized as follows. We start by describing the parser that we developed for MONGOOSE. We go on to explain why exact arithmetic is necessary for analysing metabolic networks models in a consistent and reproducible way. We describe the way we compare the results of MONGOOSE with those of COBRA [14] , a widely used metabolic network analysis tool, and CPLEX [25] , an industrial-strength linear programming solver. We continue by illustrating the structural features MONGOOSE identifies on an example network, and describing its pipeline for the structural analysis of a metabolic network. We conclude with three possible extensions to this analysis—energy balance analysis, the identification of essential and synthetic lethal reactions, and the computational design of minimal media. Description of the parser We downloaded 98 genome-scale metabolic networks representing 60 different organisms from the UCSD Systems Biology group website [17] and parsed them. The majority of the models were either provided in SBML format [35] or as Excel spreadsheets. In both cases, we performed the parsing using our own scripts in Python [36] . A few additional models provided in PDF format had to be converted into a spreadsheet format before they could be parsed. We preserved all compartment information, and considered metabolites in different compartments to be distinct, constraining them separately. We built our parser for models in SBML format on top of libSBML [37] , and the one for models in Excel spreadsheet format, on top of xlrd [38] . Because there is such a variety of formats within the latter, we had to make the parser sufficiently flexible to accommodate all of them. In addition to parsing the files, it is also able to identify a limited number of typos and other human errors introduced at the time of model generation or transcription. All the models we analysed have been extensively corrected from all the errors found by the parser, and the corrections are presented in Supplementary Table 2 . Importance of exact arithmetic Although floating-point arithmetic does not guarantee a solution that satisfies the problem constraints, there is a tolerance (defined by the linear program) that could ensure that we actually get correct results from a floating-point computation. This tolerance is the reciprocal of the largest determinant of a square submatrix of the constraint matrix A . Indeed, when a vertex is being computed, the coordinates in the basis B are determined by A B x = b B , while the others are all 0, and Cramer’s rule [22] shows that the denominator of the solution to this system equals this determinant. We note that this can be much larger than the ratio of the magnitudes of the largest and smallest entries in the constraint matrix. For instance, a Hadamard matrix of order 20 gives a ratio of 1 as all its entries are 1 or –1, but would require a tolerance of 20 −10 , or about 10 −13 . This problem of finding the largest determinant of a square submatrix of an integer matrix A turns out to be NP-hard [39] . Khachiyan [40] gives a fast approximation algorithm that gets it within a factor of m ( m /2) , where m is the number of rows of A (metabolites in the network). An alternative algorithm suggested by Michel Goemans in personal communication can approximate its logarithm within a factor of 2/5 using the fact that this logarithm can be extended to a submodular nonmonotone function on the columns of A . Unfortunately, neither of these results is practical as these estimates would require a precision of about 100 digits for a typical genome-scale metabolic network model, making calculations prohibitively slow. Comparisons to COBRA Under default settings, COBRA successfully parsed 30 models out of the 98 models we investigated, as they were written in a version of the Systems Biology Markup Language [35] matching its defaults. We did not attempt to use COBRA to parse any models in spreadsheet formats because that would have required substantial changes to many of the source files. Hence we restricted the comparison with the former models. In all our experiments, COBRA’s parameters were set to their default values, including the use of GLPK [41] as the linear program solver. By default, COBRA declares a reaction to be blocked if the minimum and maximum absolute fluxes through it are less than δ =10 −10 , while the exact arithmetic of MONGOOSE does not require any arbitrary thresholds. Comparisons with CPLEX We tested whether the structural features detected by MONGOOSE are also detected by CPLEX with its lowest feasibility tolerance of 10 −9 . We did so by creating a linear problem in CPLEX format for every feature in every metabolic network that MONGOOSE found, and tested its feasibility with CPLEX. In particular, for blocked reactions, we tested whether flux was feasible; for semiblocked reactions, we tested whether flux in the blocked direction was feasible; and for enzyme subsets, we tested whether the linear combination of the reaction fluxes could be non-zero. Out of these experiments, CPLEX was not successful with enzyme subsets, failing to identify over 100 of them in the models we tested. The results in Fig. 2 show the eight models that had the most failures, as well as the proportion of failures relative to the total number of pairs of reactions in an enzyme susbet. Although CPLEX successfully determined the blocked and semiblocked reactions in the networks we examined, we expect it to have more difficulties detecting such reactions as the size of metabolic networks continues to grow. Structural features identified by MONGOOSE Given a metabolic network with stoichiometric matrix S (reduced to contain only internal metabolites) and set of irreversible reactions , the set of admissible fluxes contains all the vectors v that satisfy the constraints A reaction i is said to be blocked if the constraints imply that v i =0. If energy balance constraints are imposed on the model, then v is an admissible flux vector if and only if where is the set of internal reactions (those not containing any extracellular metabolites). A reaction i is said to be blocked due to energy if energy balance constraints imply that v i =0. Topology-blocked reactions are an extension of the notion of dead-end reactions [14] . Although a dead-end reaction is a reaction that contains a unique internal metabolite (and is therefore constrained to have no flux to balance fluxes on that metabolite), a topology-blocked reaction is one that is revealed to be blocked in this way by the successive deletion of dead-end reactions from the network. This terminology is identical to the one used in the recent version of the sybilSBML [42] package for R [43] . In addition to orphan metabolites (ones that only participate in a single reaction), the notion of dead-end metabolite is sometimes extended to one that is only produced or only consumed; this is the definition used in the COBRA toolbox [14] . In our classification, such a metabolite would lead to a stoichiometry-blocked or an irreversibility-blocked reaction, two concepts which we discuss next. Stoichiometry-blocked reactions are reactions that are blocked only by the flux balance constraint S v = 0 . In other words, a stoichiometry-blocked reaction would be blocked even if all irreversible reactions were allowed to have flux in either direction. The corresponding notion in energy balance analysis is zero loops. Irreversibility-blocked reactions are reactions blocked by the entire set of constraints in equation (1). In other words, an irreversibility-blocked reaction would be able to have non-zero flux through it, if some or all of the irreversible reactions were allowed to have flux in either direction. The corresponding notion in energy balance analysis is energy-blocked reactions. Semiblocked reactions are those that are postulated to be reversible, but are in fact constrained by equation (1) to only admit flux in one direction, either forward ( v i ≥0) or reverse ( v i ≤0). We classify these as effectively forward or effectively reverse, depending on the allowed direction of fluxes through them. Our notion of semiblocked reactions is similar to the directionality analysis in ref. 29 , but differs from it in that it only depends on flux balance and irreversibility constraints, rather than the energy balance ones. The corresponding notion in energy balance analysis is unidirectional reactions. Enzyme subsets are maximal sets of reactions such that any steady-state fluxes in the set are in a fixed ratio. In particular, two reactions, i and j , are part of an enzyme subset if and only if there is a constant κ ≠0 such that v i = κ v j for all modes v . Each enzyme subset can be grouped together into a single reaction, which further reduces the size of the metabolic network without loss of information. The corresponding notion in energy balance analysis is isozyme subsets. In the example network below, reactions R1 and R2 are topology-blocked (note that only reaction R2 is a dead end in the sense of ref. 14 , though both are detected as such by removeDeadEnds), reactions R3 and R4 are stoichiometry-blocked, and reactions R5 through R10 are irreversibility-blocked. In addition, reactions Eno, Acn, AspC, Gdh and IlvEAvtA are semiblocked; of these, the first four are effectively forward and the last one is effectively reverse. Reactions Acn and GltA form an enzyme subset, reactions IlvEAvtA and AlaCon form another enzyme subset, and reactions Icl and Mas form a third enzyme subset. In each case, the proportionality coefficient between the fluxes is 1, consistent with the findings in ref. 19 . We note that reactions Acn and GltA are both irreversible, as are reactions IlvEAvtA and AlaCon; it is always the case that the reactions in each subset are either all irreversible (with positive proportionality coefficients) or all reversible, provided that the semiblocked reactions have been properly adjusted, as we show in Methods. Finally, the flux balance constraints on A through G, as well as on metabolites Ala, Cit, CoA and Gly are deleted as redundant. This reduces the example network from an initial size of 23 × 34 to a final size of 12 × 21. Example network: internal metabolites: A, B, C, D, E, F, G; AcCoA, Ala, Asp, Cit, CoA, Fum, Glu, Gly, IsoCit, Mal, OAA, OG, PEP, Pyr, Succ, SucCoA. external metabolites: ADP, Alaex, AMP, Aspex, ATP, CO2, FAD, FADH2, Gluex, NAD, NADH, NADP, NADPH, NH3, PG, Sucex. reactions: Description of the MONGOOSE pipeline MONGOOSE performs all its computations using the fractions module available in versions 2.6 and higher of Python [36] . All linear optimizations are performed with the QSopt_ex solver [23] , which uses the simplex algorithm [44] and tests solution optimality in exact arithmetic. The rational dual variables output by the solver provide a certificate for the correctness of the solution to our linear optimization problems and can be verified independently of the solver. The MONGOOSE pipeline begins by converting an input metabolic model (in the form of a stoichiometric matrix) into canonical form. A canonical form of a stoichiometric matrix contains just the right amount of information needed to perform further analysis, the results of which can then be post-processed to obtain results for the original network. Formally, a matrix is said to be in canonical form if it contains no blocked reactions, unidirectional reactions (reversible reactions which can only proceed in the forward or only in the reverse direction) or enzyme subsets, and has linearly independent rows. Below we describe each step of the process for reducing a network to its canonical form. A reaction is said to be blocked if it cannot have non-zero flux in any mode. We propose to classify blocked reactions by the cause of blockage. Recall from the previous subsection that reaction i is topology-blocked if it contains a metabolite not participating in any other reaction, stoichiometry-blocked if S v = 0 implies that v i =0, or irreversibility-blocked if equation (1) implies v i =0. Since topology-blocked reactions are also stoichiomety-blocked, and stoichiomety-blocked reactions are also irreversibility-blocked, we use the simplest cause of blockage that applies in our classification. Topology-blocked reactions are readily identified by a simple analysis of the number of reactions each metabolite is involved in. Stoichiometry-blocked reactions can be identified in a fully reversible network S by performing a Gauss–Jordan elimination on S to find rows with a unique 1 in them, while irreversibility-blocked reactions in a fully irreversible network can be identified by the algorithm given in Supplementary Note 3 . It is surprising that algorithms guaranteed to work only on a fully reversible and a fully irreversible network respectively can be combined to work on a general network. Nevertheless, the simple algorithm consisting of a sequential application of these two algorithms turns S into a consistent matrix by deleting all its blocked reactions, as shown in Supplementary Note 4 . We call a reversible reaction unidirectional if it can sustain a flux of only one sign. If this sign is positive, we call the reaction effectively forward, whereas if it is negative, we call it effectively reverse. To decide whether a reversible reaction i is unidirectional, it suffices to test the feasibility of two linear programs, one with v i =1 and one with v i =–1. Since S is now a consistent matrix, at least one of those will always be feasible. Once all unidirectional reactions have been identified, we reverse the effectively reverse reactions by multiplying all their coefficients in S by –1, and then add all the unidirectional reactions to . Supplementary Note 5 shows that all the enzyme subsets can be identified from the proportional columns of the nullspace matrix K of S . Hence, the algorithm given by Gagneur and Klamt [10] correctly identifies all such subsets (something that was not known before the structural results presented here). Furthermore, since S no longer has any unidirectional reactions, any enzyme subset will consist either only of irreversible reactions or only of reversible reactions. If an enzyme subset containing reactions i 1 , i 2 ,…, i t has been identified, let r j be the ratio of the flux through i j to the flux through i 1 , for 2≤ j ≤ t . We can then lump the enzyme subset together into a single new reaction (here, subscripts indicate matrix columns). This significantly reduces the size of S without losing any information, since any mode in the compressed matrix can be expanded back to a mode in the original matrix [10] . After we make S consistent, deal with the unidirectional reactions and lump together the enzyme subsets, we can remove the redundant constraints (rows that are linear combinations of other rows) by Gaussian elimination on S T . Each of these corresponds to a conservation relation among the metabolites in the network [45] . Unlike the reduction process described by Gagneur and Klamt [10] , the reduction process that we propose here is guaranteed to converge after one iteration ( Supplementary Note 6 ). The resulting matrix is said to be in canonical form. Once the matrix is in canonical form, it may be necessary to unblock its biomass reaction. If the biomass reaction is topology-blocked, this indicates an incompleteness in the model (one of the biomass components cannot be produced). If it is stoichiometry-blocked, it can be unblocked by removing balance constraints from a small subset of metabolites. This subset of metabolites can provide clues in a rational search for missing reactions. Finding the smallest such subset is NP-hard [12] ; however, a small subset can be found by a linear program based on the key observation that we can look for vectors v with v biomass =1 such that S v has small support. If the biomass reaction is irreversibility-blocked due to the directional restrictions on some reactions, it can be unblocked by making a small subset of the irreversible reactions reversible. As above, finding the smallest such subset is NP-hard, but a small subset can be found by a linear program. Indeed, here we look for a vector v such that S v = 0 with v biomass =1 and few components of v are negative, which by Supplementary Note 3 is equivalent to finding a small cutset for the biomass reaction in the nullspace matrix of S . Once the stoichiometric matrix is in canonical form and its biomass reaction has been unblocked if necessary, further queries can be performed on the metabolic model as described in the following subsections. Energy balance analysis The energy balance constraints on a network with stoichiometric matrix S and internal reactions are given by equation (2). Similarly to FBA, energy balance analysis constraints can be used to reduce the model and identify its structural features, with the key difference that instead of applying to the nullspace of the entire stoichiometric matrix S , the constraints apply to the row space of , the part of the stoichiometric matrix containing the internal reactions. The structural analysis and reduction proceed analogously to FBA, with the key difference that unlike the nullspace of S , for which a basis must be constructed via a Gauss–Jordan elimination, the row space of is given explicitly by the model. Once the analysis is completed, the reduced version of is merged back with the external reactions in S , and it is at that stage that any redundant constraints are eliminated. The final stage of the analysis involves finding restrictions on the signs of the flux vectors. This task can be accomplished by finding all the elementary flux modes of the network containing only the internal reactions [29] . While this is a computationally intractable problem, Supplementary Note 8 shows that this analysis can be performed on the fully reduced network, rather than the original network, without loss of information. Essential and synthetic lethal reactions In a metabolic model, a reaction is predicted to be essential if disabling it blocks the biomass reaction. To find all such reactions, we first compute some modes involving the biomass reaction, and then test those reactions that are active in each of those modes for essentiality. To test whether a reaction i is essential, we check whether the biomass reaction can be active when equation (1) holds with v i =0. Note that every reaction in an enzyme subset with the biomass reaction is automatically essential. To find all the remaining ones, we generate a short flux mode u in the reduced network such that u biomass =1 by minimizing the 1-norm of u , and then check essentiality of each reaction i active in u by checking for feasibility of equation (1) with v i =0 and v biomass =1. In this way, for each i , we obtain a certificate of essentiality or a vector v with v i =0 and v biomass =1. A pair of reactions is called synthetic lethal if neither of them is essential, but disabling both of them disables growth. To compute all pairs of synthetic lethal reactions, we use the vector u from the previous step together with the vectors v corresponding to each nonessential reaction i active in u . Let L be the number of such vectors. Let G denote the set of nonessential reactions active in at least one of these vectors. We construct a matrix M of size | G | with M i , j being the number of modes that contain both i and j , with the diagonal element M i , i being the number of vectors that contain reaction i . The pair { i , j } is synthetic lethal for the L vectors if and only if each one of them contains either i or j , which is to say that M i , i + M j , j − M i , j = L , so we only check pairs satisfying this condition. This leads to a substantial reduction in the number of checks. Minimal media A minimal medium is a minimal subset of the exchange reactions that can sustain the organism’s growth. The problem of finding all minimal media is NP-hard, and has been studied previously [11] . MONGOOSE can identify a number of small minimal media as follows. It starts by finding a vector v satisfying equation (1) with v biomass =1 that minimizes the sum of components corresponding to . This is a minimal medium. At each subsequent step, constraints are introduced to steer the solution away from any previously found ones. More specifically, if we denote by R ( v ) the set of non-zero components of v , a minimal medium v uniquely minimizes ∑ j ∉ R ( v ) v j with a value of 0. It can be shown that the medium with the second-best value, u , will be a linear combination of v and another minimal medium w , if an active-set algorithm [46] such as the simplex algorithm [44] is used. u can be found by solving the linear program for some small number ε >0. Once u is found, we can simply subtract the largest multiple of v that still keeps it nonnegative, and this will be w . The same procedure can now be repeated starting from w instead of v . This procedure continues until no new minimal medium is found. How to cite this article: Chindelevitch, L. et al. An exact arithmetic toolbox for a consistent and reproducible structural analysis of metabolic network models. Nat. Commun. 5:4893 doi: 10.1038/ncomms5893 (2014).